Enzymatic aerobic ring rearrangement of optically active furylcarbinols Biogenic furans are currently discussed as highly attractive alternative feedstock in a post-fossil society; thus, also the creation of sustainable furan valorization pathways appears of great importance. Here an artificial Achmatowicz monooxygenase activity for the aerobic ring expansion of furans is achieved by the combination of commercial glucose oxidase as oxygen-activating biocatalyst and wild-type chloroperoxidase as oxygen-transfer mediator, providing a biological ready-to-use solution for this truly synthetic furan rearrangement. In concert with enzymatic transformations for the enantioselective preparation of optically active furylcarbinols, purely biocatalytic reaction cascades for the stereocontrolled construction of complex pyranones are obtained, exhibiting high functional group tolerance even to oxidation-sensitive moieties. In the course of the inevitable medium- to long-term reorganization of our value chains from fossil resources towards a general supply on the basis of renewable raw materials, one of the great challenges in the near future will comprise the development of novel processes and the adaptation of existing synthetic strategies to those new requirements. Currently, biogenic furans, obtained through biorefinery of lignocellulose, are considered one of the most promising core structures among the plant-based, non-edible raw material platforms [1] . While the energetic use of renewables has to be met with a certain scepticism not only from a chemist’s perspective [2] , [3] , the role of biomolecules as rich source of green synthetic building blocks is far less controversially discussed. In addition to defunctionalization routes from biogenic furans to structurally simple base chemicals [4] , [5] , [6] , this heterocyclic moiety offers an interesting repertoire of unique rearrangement reactions, providing pathways for the generation of complex molecular architectures [7] , [8] , [9] , [10] . The oxidative ring expansion of α-heterofunctionalized furans according to Achmatowicz represents a role model in this perspective [10] , opening up an elegant access to densely decorated pyran- ( Fig. 1a ) as well as piperidine derivatives [11] . First mentioned already in 1971, various ways to substitute elemental bromine by other oxidative agents were investigated with the result that today a multitude of modern procedures for the selective furan cleavage are available [12] , [13] , [14] , [15] , [16] . However, with the rapidly increasing number of applications of Achmatowicz’s oxidation in complex synthetic scenarios, it remains to be noted that classical oxidants such as 3-chloroperbenzoic acid and N -bromosuccinimide still represent the means of choice [17] , [18] , [19] . 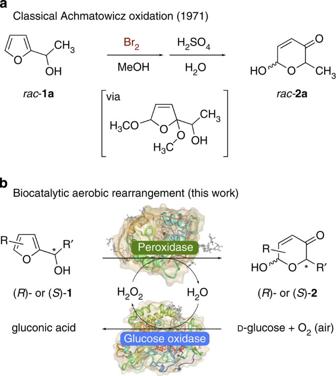Figure 1: Oxidative ring expansion of furylcarbinols: historical precedent and modern interpretation. (a) Formation of 2,5-dimethoxy-2,5-dihydrofuran on oxidation with bromine in methanol is followed by acetal cleavage and ring expansion via an intermediate 4-ketoenal. (b) Schematic representation of the coupled biocatalytic Achmatowicz rearrangement combining aerobic reduction of oxygen by glucose to hydrogen peroxide with the peroxidase-mediated oxygen transfer onto the furan core. Figure 1: Oxidative ring expansion of furylcarbinols: historical precedent and modern interpretation. ( a ) Formation of 2,5-dimethoxy-2,5-dihydrofuran on oxidation with bromine in methanol is followed by acetal cleavage and ring expansion via an intermediate 4-ketoenal. ( b ) Schematic representation of the coupled biocatalytic Achmatowicz rearrangement combining aerobic reduction of oxygen by glucose to hydrogen peroxide with the peroxidase-mediated oxygen transfer onto the furan core. Full size image In the light of a sustainable utilization of biogenic building blocks, the development of environmentally benign valorization pathways has to be regarded a paramount task, and in our opinion, biological catalysts have to be considered most suitable to fulfil these requirements. However, biocatalysis is hampered by one simple factor, that is, the lack of biosynthetic precedence for a variety of synthetically relevant transformations and the consequent lack of natural catalysts to promote the desired reactions. Thus, the identification of promiscuous activities by wild-type enzymes as well as the evolution of new reactivities with the aid of biotechnological and chemical tools are highly warranted [20] , [21] , [22] . In this report, we disclose an unprecedented, purely enzymatic protocol for the non-natural Achmatowicz-type rearrangement of furylcarbinols employing an oxygen activation cascade based on commercially available biocatalysts ( Fig. 1b ). Our experimental design rests on the initial finding of selective oxygen-transfer abilities of peroxidases in the oxidative ring expansion of substituted furfuryl alcohols. The linkage with a hydrogen peroxide-evolving system based on the bioreduction of aerial oxygen by cheap and ecologically benign biomolecules such as glucose renders a fully integrated, highly practicable and sustainable protocol allowing for the rearrangement not only of simple carbinols but likewise for a series of real-world substrates carrying synthetically versatile functional groups. Catalyst identification Owing to the absence of Achmatowicz-like transformations in biosynthesis, studies on the furan metabolism in mammals served as foundation for our development of a synthetic enzyme-based protocol. Toxicokinetic studies on pulegone and menthofuran detoxification pathways by Nelson and co-workers [23] did not only identify human liver cytochrome P450 monooxygenases as catalysts involved in furan degradation, but also provided evidence for the formation of furanoepoxides, which is also expected in the chemical Achmatowicz oxidation by electrophilic oxygenation agents. Thus, as robust and relatively cheap functional mimics of cytochrome P450s [24] , four haem-based peroxidases were evaluated on their potential to catalyse the selective oxidation of furylcarbinol rac - 1a to give the ring-expanded product rac - 2a . With gluconate as sole carbon-based side product, commercial glucose oxidase ( Aspergillus niger , GOx) was chosen as a release system for hydrogen peroxide through the catalytic reduction of aerial oxygen, offering the benefits of simple product separation and an excellent ecological profile [25] , [26] . In the absence of potential oxygen-transfer catalysts as well as in the presence of soybean peroxidase ( Table 1 , entry 1), no conversion was observed and rac - 1a was recovered quantitatively after 2 days of incubation. In contrast, using bovine lactoperoxidase or horseradish peroxidase ( Table 1 , entries 2 and 3), slow consumption of the furylcarbinol was detected and in the latter case, traces of the Achmatowicz product rac - 2a were isolated after 48 h. An entirely different picture was drawn implementing chloroperoxidase from Caldariomyces fumago (CPO) into the system [27] . Sometimes referred to as peroxidase–cytochrome P450 functional hybrid, CPO shares structural properties with P450 enzymes such as a thiolate as axial haem ligand explaining a much more diverse reaction portfolio compared with other peroxidases including effective cytochrome-like oxygen-transfer processes [28] . Within 2 h, full conversion of rac - 1a was achieved and the desired pyranone rac - 2a could be isolated in 51% yield ( Table 1 , entry 4). As pH variation did not result in any improvement of the catalytic system ( Supplementary Fig. 1 ), we turned our attention to potentially beneficial effects of cosolvents ( Supplementary Fig. 2 ). Here, polar additives (10% v/v) like dimethylsulfoxide, acetonitrile ( Table 1 , entries 5 and 6) or acetone reduced the rates of oxidation. On the other hand, in two-phase systems based on hydrophobic solvents (toluene, heptane, ethyl acetate) the oxidative ring expansion did not take place at all. In strong contrast, in the presence of tert -butanol as cosolvent, not only the enzymes’ activity was well conserved but more importantly, product rac - 2a could be isolated in substantially higher yield of 82% ( Table 1 , entry 7). While the addition of t BuOH had only marginal effect on the rate of furan consumption, the boost in yield can rather be attributed to considerably enhanced product stability with a half-life of pyranone 2a of 40.7 h (±3.7 h) as compared with 11.9 h (±0.2 h) in the purely aqueous medium ( Supplementary Fig. 3 ). In addition, we could prove that also other hydrogen peroxide-evolving systems such as L -leucine/ L -amino-acid oxidase ( Crotalus atrox ) support the CPO-catalysed rearrangement; however, due to the significantly higher cost of the enzymes and lower reaction rates, these alternatives were not further pursued ( Supplementary Fig. 4 ). Moreover, a single-enzyme approach was studied where hydrogen peroxide was slowly added by syringe pump to a buffered solution of rac - 1a and CPO. In this case, full conversion was achieved after 2 h and rac - 2a could be isolated in 67% yield ( Table 1 , entry 8). Table 1 Oxidase/peroxidase-mediated oxidation of rac -1-(2-furyl)ethanol. Full size table Mechanistic considerations With the identification of the GOx/chloroperoxidase couple as efficient system for the aerobic Achmatowicz oxidation, questions about the underlying functional principle arose. As the native functions of haloperoxidases include the oxidation of halides to hypohalites [29] , [30] , the initial goal was to shed light on whether a halide/hypohalite mediator system qualified as final oxidizing species or rearrangement was induced through direct substrate–enzyme interaction and oxygen transfer from the prosthetic oxidized haem unit (compound I). First studies revealed that incubation of rac - 1a in a buffered NaOCl solution in the absence of potential catalysts led indeed to oxidative ring expansion to give traces of pyranone rac - 2a ; however, reaction rates substantially lagged behind the GOx/CPO-catalysed transformation. Furthermore, considerable inhibition of the enzymatic rearrangement was observed in chloride-containing reaction media (half-maximal inhibitory concentration=7.4 mM; Supplementary Fig. 5 ). Another obvious evidence for a direct interaction between substrate and chloroperoxidase resulted from the time-dependent stereochemical analysis of the GOx/CPO-mediated reaction of rac - 1a . At low conversion, a distinct kinetic resolution with an enantioselectivity of E =4.5 was observed ( Fig. 2a ), implying at least the participation of a protein-bound oxidizing species. The strongest indication for the non-mediated furan oxidation through compound I, or alternatively through a hydroperoxoferric intermediate [31] , arose from experiments using isotopically labelled oxygen as terminal oxidant [32] . Ring expansion by the GOx/CPO system in an argon atmosphere enriched in heavy oxygen (20 vol% 18 O 2 ) gave rise to the mono- 18 O-marked product rac - 2a - 18 O in high isotopic yield ( Fig. 2b ). Moreover, mass spectrometric fragment analysis disclosed a low degree of regioselectivity in the oxygen transfer onto the furan core with a slight preference for the less-substituted position ( Supplementary Fig. 6 ) [33] . Determination of the kinetic parameters for the aerobic oxidation of rac - 1a revealed an apparent turnover frequency of the peroxidase of k cat =370.7 min −1 (±9.3 min −1 ) and a good affinity for this non-natural substrate of K M =141 μM (±27 μM) with a total turnover number of ~121,400 at 50 mM substrate concentration ( Supplementary Fig. 7 ). In addition, the hypothesis of oxygen transfer from the oxidized prosthetic group was strongly supported by fundamental experiments on a redox-neutral enzymatic rearrangement. Oxygen-transfer-based redoxisomerization of hydroperoxide rac - 3a by chloroperoxidase from C. fumago as sole catalyst did not only proceed smoothly, coincubation with equimolar amounts of the deuterium-labelled alcohol rac - 1a - d 3 yielded the Achmatowicz product 2a alongside with only minor amounts of the CD 3 -marked pyranone 2a - d 3 . While indicating that initial reduction of the hydroperoxide and reoxidation of the so-formed furylcarbinol take place in a coupled manner without diffusion as dominant pathway ( Fig. 2c ; Supplementary Fig. 8 ), this experiment also clearly refutes working hypotheses about non-haem or ferric oxidizing species. Moreover, also the use of t -butyl hydroperoxide as external oxidizing agent proved to be effective ( k cat =98.8 min −1 (±28.1 min −1 )) and led to the formation of 2a from alcohol 1a in the presence of chloroperoxidase, ruling out alternative reaction pathways such as formation and consequent reduction of endoperoxide intermediates. On the basis of these results, we propose that the biocatalytic Achmatowicz-type rearrangement by chloroperoxidase proceeds via oxygenation [23] , [34] of the furan core through oxygen transfer from an oxoferryl porphyrin species and subsequent ring fission and recyclization to give the pyranone products ( Supplementary Fig. 9 ). 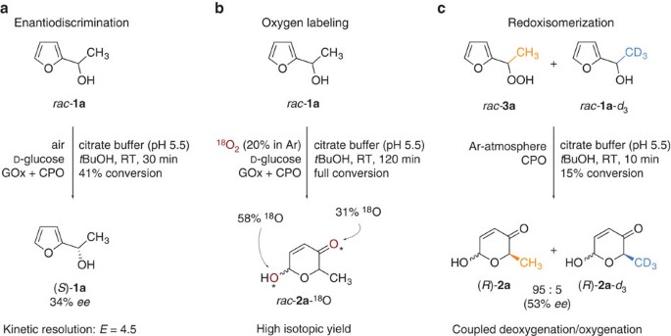Figure 2: Indications for the direct peroxidase–furan interaction. (a) Conversion of racemic furylethanol by chloroperoxidase is accompanied by enrichment of the (S)-alcohol through kinetic resolution (krel=4.5). (b) Incorporation of18O by incubation under18O2-enriched argon atmosphere. (c) Coincubation of furylhydroperoxide and furylcarbinol in the absence of external oxidizing agents leads to selective formation of the hydroperoxide-derived product. The reaction was stopped at low conversion to deliberately overestimate1a/1a-d3-scrambling as expected for a potential alcohol diffusion pathway. Figure 2: Indications for the direct peroxidase–furan interaction. ( a ) Conversion of racemic furylethanol by chloroperoxidase is accompanied by enrichment of the ( S )-alcohol through kinetic resolution ( k rel =4.5). ( b ) Incorporation of 18 O by incubation under 18 O 2 -enriched argon atmosphere. ( c ) Coincubation of furylhydroperoxide and furylcarbinol in the absence of external oxidizing agents leads to selective formation of the hydroperoxide-derived product. The reaction was stopped at low conversion to deliberately overestimate 1a / 1a- d 3 -scrambling as expected for a potential alcohol diffusion pathway. Full size image Towards coupled multi-enzymatic processes Even if a certain extent of stereoselectivity was observed in the oxidative transformation of rac - 1a , the low degree of enantiodiscrimination would not allow for a preparatively reasonable kinetic resolution of this substrate. As kinetic resolutions exhibit the general flaw of yield limitation, our aim was to synthesize optically active furylcarbinols via preceding biotransformations to subsequently rearrange them on the basis of the artificial Achmatowicz monooxygenase system. The asymmetric reduction of the corresponding furylketones ( 3a – k ) through alcohol dehydrogenases (ADHs) proved to be an efficient and convenient method [35] , [36] . Two commercial ADHs in a substrate-coupled system with isopropanol as terminal reducing agent enabled the preparation of alcohol 1a whereby, depending on the employed ADH, both ( R )- 1a and ( S )- 1a were obtained in nearly enantiopure form. The succeeding GOx/CPO-mediated aerobic rearrangement to the pyranones ( R )- 2a and ( S )- 2a , respectively, proceeded in good yield, with quantitative preservation of optical activity and without perceptible matched/mismatched effects ( Table 2 ). Employing the anti-Prelog-selective ADH, various ketones were reduced in high enantioselectivity and subsequently subjected to the aerobic biocatalytic rearrangement. Oxidative ring expansion of the enantiomerically enriched ethyl- and propyl-substituted alcohols 1b and 1c and even of the sterically encumbered isopropylcarbinol 1d succeeded in good yield. Moreover, the CPO-catalysed transformation of the alcohols 1c (95% ee ) and 1d (97% ee ) was accompanied by further increase in optical purity of the pyranone products (≥98% ee ). The extent of enantiodiscrimination of CPO towards substrate 1d was determined in an oxidative kinetic resolution with a relative rate of k rel =9.6. Hence, with regard to a broader substrate tolerance in both enantiomeric series, evolution of less-stereoselective chloroperoxidases appears desirable in the longer run. Apart from that, a high functional group tolerance of CPO could be illustrated in the rearrangement of the alcohols 1e – h . Not only substrates such as chlorohydrine 1e or β-hydroxyester 1f smoothly rearranged in the presence of the GOx/CPO system to give the pyranones 2e (64%) and 2f (68%), respectively, more gratifyingly, even oxidation-sensitive elements like olefins ( 2g , 65%) and primary alcohols ( 2h , 31%) were well tolerated by the peroxidase. Solely, oxidation of the propargylic alcohol 1i turned out problematic and the corresponding rearrangement product could not be isolated. With the use of core-substituted furylcarbinols, a structural limitation became apparent. While biocatalytic reduction of the 5-substituted furylketones gave rise to the enantiopure alcohols 1j and 1k , their oxidative ring expansion failed even with prolonged reaction time and substantially increased enzyme loadings. Table 2 Biocatalytic Achmatowicz rearrangement of optically active furanols. Full size table Since both the asymmetric ketone reduction for the construction of enantioenriched furylcarbinols as well as their oxidative rearrangement could potentially be attained on the basis of glucose-dependent biotransformations, it seemed logical to strive after a direct linkage of both reactions to establish a multi-enzyme cascade for the synthesis of optically active Achmatowicz products. Essentially, pyranone ( R )- 2a could be detected in traces in a genuine four-enzyme/one-pot reaction; however, much more satisfying results were obtained by sequential addition of the individual catalysts and concurrent pH adjustment. Thus, after reaching nearly full conversion of the ketone 4a by a glucose dehydrogenase (GDH)/ADH system, the reaction mixture was slightly acidified. With the addition of GOx and chloroperoxidase, fast and selective formation of the pyranone was observed ( Supplementary Fig. 10 ) and ( R )- 2a was isolated in 47% yield and >99% ee ( Fig. 3 ). In a triple catalytic system, where the GDH-mediated cofactor recycling was replaced by the previously employed dehydrogenation of isopropanol, the same one-pot principle provided ( R )- 2a in enantiopure form and 59% yield. 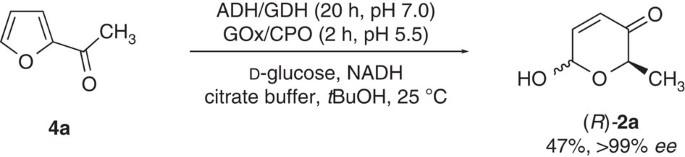Figure 3: Combination of two glucose-dependent biotransformations: four enzymes—two steps—one pot. The reaction was performed in a sequential manner due to incompatible pH optima of the individual catalytic systems. SeeSupplementary Methodsfor full experimental details. Figure 3: Combination of two glucose-dependent biotransformations: four enzymes—two steps—one pot. The reaction was performed in a sequential manner due to incompatible pH optima of the individual catalytic systems. See Supplementary Methods for full experimental details. Full size image Diffusible redox mediators to overcome structural limitations Although excellent selectivities, sustainable reaction conditions and high functional group tolerance of the presented Achmatowicz system leave no doubt that this novel application represents a valuable extension of the existing biocatalytic portfolio, our delight was marginally tempered by its limitation to monosubstituted furans. Directed evolution of the biocatalyst with regard to an extended substrate spectrum seems to be a logical next step to address this issue [37] . From the chemist’s perspective, however, also the reconstruction of the catalytic system’s architecture by allowing for non-protein-bound diffusible oxygen-transfer mediators appeared as an attractive alternative to eliminate undesired substrate effects. In search of suitable redox mediators combining activity in the furan oxidation with the disability to oxidize secondary alcohols, our choice fell on peracetic acid. Perhydrolysis of carboxylic acid derivatives through lipases and utilization of the so-formed peracids in oxidation reactions represents a well-studied approach [38] , [39] . In analogy to the oxidase/peroxidase couple, we aimed for the concatenation of the biocatalytic reduction of aerial oxygen with the activation of hydrogen peroxide by enzymatic peracetate formation. The combination of GOx with a lipase from Candida antarctica (type B, non-immobilized preparation) in acetate buffer at pH 4.5 proved to be a viable catalytic system for the selective aerobic oxidation of rac - 1j , as the 2,6-dimethylated pyranone 2j was produced in moderate yield ( Fig. 4 ). Even if substantially prolonged reaction times and the unfavourable optimum pH with regard to configurational lability of the furylcarbinols (see Supplementary Fig. 11 , for racemization under acidic conditions) unquestionably demand vernier adjustments of this biocatalytic Achmatowicz variant, the application of diffusible, yet selective mediators might mature to an auspicious and practical alternative to the direct oxidation by haem-based enzymes. 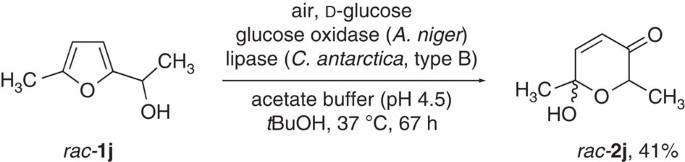Figure 4: Aerobic Achmatowicz oxidation of 2,5-disubstituted furans. On the basis of the enzyme cascade consisting of an oxidase and a lipase, peracetic acid is formed catalytically from the acetate buffer that can act as diffusible redox mediator in the oxidation of otherwise non-reactive furylcarbinols. Figure 4: Aerobic Achmatowicz oxidation of 2,5-disubstituted furans. On the basis of the enzyme cascade consisting of an oxidase and a lipase, peracetic acid is formed catalytically from the acetate buffer that can act as diffusible redox mediator in the oxidation of otherwise non-reactive furylcarbinols. Full size image Over the years, biocatalysis has made its way into synthetic organic chemistry; however, in most cases, the role of enzymatic transformations is limited to the supply of non-racemic small-molecule building blocks with only marginal-to-non-existing contribution to the creation of molecular complexity. Herein, we demonstrated the use of biocatalysts outside their natural setting, tackling a non-natural rearrangement reaction converting structurally simple and readily available furylcarbinols into high-value synthetic building blocks in a preparatively convenient and eco-friendly manner. Aiming for the valorization of biogenic furans, future investigations will expand towards biological cascades for the direct conversion of lignocellulose-derived furfurals by means of lyases as well as the construction of combined organo-/biocatalytic reaction sequences. With the recent advances in biotechnological process development, there is a true potential to design fermentation pathways implementing further optimized peroxidases or monooxygenases for selective Achmatowicz-type rearrangements that would allow for integrated furan refinement up the ladder of molecular complexity also in a more technical context. General methods Commercially available reagents were used without further purification. 18 O 2 (98 atom%) was purchased from Carbolution Chemicals GmbH. Catalysts and cofactors were obtained from: NADH, Carbolution Chemicals GmbH; chloroperoxidase from C. fumago ( CPO ), 21.9 kU ml −1 , Bio-Research Products; GOx type II ( GOx ), 17.3 U mg −1 , Sigma; ADH, recombinant from Escherichia coli ( ADH 200 ), 17.6 U mg −1 , evocatal GmbH; ADH, recombinant from E. coli ( ADH 030 ), 18.8 U mg −1 , evocatal GmbH; and glucose dehydrogenase, recombinant from E. coli ( GDH 060 ), 214 U mg −1 , evocatal GmbH. Presented data are average numbers of at least two replicate experiments. All products were purified by column chromatography over silica gel (Macherey-Nagel MN-Kieselgel 60 (40–60 μm, 240–400 mesh)). Analytical thin-layer chromatography was performed on Macherey-Nagel precoated silica gel plates (ALUGRAMM Sil G/UV254). 1 H- and 13 C-NMR spectra were recorded on a Bruker Avance 300 spectrometer at room temperature at 300 and 75 MHz, respectively. Chemical shifts are reported in parts per million (p.p.m.) relative to tetramethylsilane. Infrared spectra were recorded on a Shimadzu IRAffinity-1 Fourier transform infrared (FTIR) spectrometer, absorption bands were reported in wave numbers (cm −1 ). Gas chromatography was performed on a Hewlett Packard HP 6890 Series GC System using a Macherey-Nagel FS-Lipodex A and Macherey-Nagel FS-Lipodex E column (25 m × 0.25 mm), N 2 , 1.0 ml min −1 ; method A: 50 °C (1 min)/5 °C min −1 (35 min)/120 °C (15 min); method B: 40 °C (5 min)/2 °C min −1 (10 min)/5 °C min −1 (50 min). High-performance liquid chromatography was performed on a Merck D-7000 with a Merck L-4500 PDA detector using an analytical Daicel Chiralpak column (250 × 4.6 mm). Optical rotations were measured on a Perkin-Elmer 343plus. For full experimental details, see Supplementary Methods . Biocatalytic Achmatowicz rearrangement In a 100-ml round bottom flask, furylcarbinol ( R )- 1f (99% ee , 10 mM, 0.5 mmol) was dissolved in a mixture of citrate buffer (45 ml, 100 mM, pH 5.5) and t -butanol (5 ml). After addition of chloroperoxidase (0.41 μM, 0.5 kU), GOx (3.6 μM, 0.5 kU) and D -glucose (50 mM), the solution was incubated (room temperature, 500 r.p.m.) for 120–180 min. L -Methionine (250 mg) was added and the reaction mixture was extracted with ethyl acetate (3 × 15 ml). The combined organic layers were dried over MgSO 4 , evaporated under reduced pressure and (2 R )-6-hydroxy-2-(ethoxycarbonylmethyl)-2H-pyran-3(6H)-one ( 2f ) was obtained after column chromatographic purification (SiO 2 , cyclohexane/ethyl acetate, 4/1) as colourless oil (68.1 mg, 0.34 mmol, 68%, α / β =72/28). : +7.4 (c 1.00, CHCl 3 ), 99% ee . R f (cyclohexane/ethyl acetate, 2/1): 0.19. α- 2f : 1 H-NMR (300 MHz, CDCl 3 ): δ (p.p.m. )=6.93 (dd, 3 J =10.3 Hz, 3 J =3.5 Hz, 1H), 6.17 (d, 3 J =10.3 Hz, 1H), 5.75–5.53 (m, 1H), 5.03 (dd, 3 J =7.2 Hz, 3 J =4.0 Hz, 1H), 3.00–2.98 (m, 1H), 2.85–2.68 (m, 1H), 1.30–1.25 (m, 3H); 13 C-NMR (75 MHz, CDCl 3 ): δ (p.p.m. )=195.0, 171.0, 144.6, 127.1, 87.4, 70.7, 61.0, 35.3, 14.1. β- 2f (selected signals): 1 H-NMR (300 MHz, CDCl 3 ): δ (p.p.m. )=6.98 (dd, 3 J =10.3 Hz, 3 J =1.5 Hz, 1H), 6.13 (dd, 3 J =10.3 Hz, 3 J =1.5 Hz, 1H), 4.61–4.57 (m, 1H), 4.21–4.13 (m, 3H), 3.06–3.03 (m, 1H); 13 C-NMR (75 MHz, CDCl 3 ): δ (p.p.m. )=194.4, 171.0, 148.4, 128.4, 90.9, 75.3, 67.4, 36.2, 14.1. FTIR (neat, ATR): ν (cm −1 )=3420 (br), 2988 (w), 1732 (m), 1693 (m), 1375 (w), 1286 (w), 1178 (m), 1089 (m), 1020 (s), 931 (w), 846 (w), 759 (w). Coupled one-pot reduction rearrangement ADH (5.7 mg, 0.1 kU, ADH 200 ), glucose dehydrogenase (1.4 mg, 0.3 kU, GDH 060 ) and D -glucose (100 mM) were added to a solution of acetylfuran ( 4a , 18.5 mM, 110 mg) and NADH (1.8 mM) in phosphate buffer (54 ml, 50 mM, pH 7.0) and the mixture was incubated for 24 h (25 °C, 500 r.p.m.). Citric acid was added to adjust the pH to 5.5. After further addition of t -butanol (5 ml), chloroperoxidase (0.35 μM, 0.5 kU), GOx (3.0 mM, 0.5 kU) and D -glucose (40 mM), the solution was incubated for 180 min (25 °C, 500 r.p.m.). L -Methionine (250 mg) was added and the reaction mixture was extracted with ethyl acetate (3 × 15 ml). The combined organic layers were dried over MgSO 4 , evaporated under reduced pressure and the (2 R )-6-hydroxy-2-methyl-2H-pyran-3(6H)-one ( 2a ) was obtained after column chromatographic purification (SiO 2 , cyclohexane/ethyl acetate, 5/1) as colourless solid (60.1 mg, 0.47 mmol, 47%, α / β =67/33). : −79.6 (c 0.50, CHCl 3 ), 99% ee. Melting point: 61 °C. R f (cyclohexane/ethyl acetate, 2/1): 0.25. α- 2a : 1 H-NMR (300 MHz, CDCl 3 ): δ (p.p.m. )=6.89 (dd, 3 J =10.2 Hz, 3 J =3.2 Hz, 1H), 6.10 (d, 3 J =10.2 Hz, 1H), 5.63 (m, 1H), 4.71 (q, 3 J =6.7 Hz, 1H), 3.53 (d, 3 J =5.0 Hz, 1H), 1.38 (d, 3 J =6.7 Hz, 3H); 13 C-NMR (75 MHz, CDCl 3 ): δ (p.p.m. )=197.0, 144.5, 127.3, 87.7, 70.4, 15.3. β- 2a : 1 H-NMR (300 MHz, CDCl 3 ): δ (p.p.m. )=6.94 (d, 3 J =10.2 Hz, 1H), 6.15 (d, 3 J =10.2 Hz, 1H), 5.67 (d, 3 J =7.2 Hz, 1H), 4.23 (1H, m), 3.87 (d, 3 J =7.2 Hz, 1H), 1.45 (d, 3 J =6.7 Hz, 3H); 13 C-NMR (75 MHz, CDCl 3 ): δ (p.p.m. )=196.5, 148.1, 128.6, 91.0, 75.3, 16.2. FT-IR (neat, ATR): ν (cm −1 )=3294 (br), 3051 (w), 2987 (w), 1676 (s), 1435 (m), 1371 (m), 1334 (w), 1273 (w), 1232 (m), 1143 (m), 1109 (m), 1091 (m), 1031 (s), 937 (m), 900 (m), 808 (m), 690 (m). How to cite this article: Thiel, D. et al . Enzymatic aerobic ring rearrangement of optically active furylcarbinols. Nat. Commun. 5:5278 doi: 10.1038/ncomms6278 (2014).